miR-137 forms a regulatory loop with nuclear receptor TLX and LSD1 in neural stem cells miR-137 is a brain-enriched microRNA. Its role in neural development remains unknown. Here we show that miR-137 has an essential role in controlling embryonic neural stem cell fate determination. miR-137 negatively regulates cell proliferation and accelerates neural differentiation of embryonic neural stem cells. In addition, we show that the histone lysine-specific demethylase 1 (LSD1), a transcriptional co-repressor of nuclear receptor TLX, is a downstream target of miR-137. In utero electroporation of miR-137 in embryonic mouse brains led to premature differentiation and outward migration of the transfected cells. Introducing a LSD1 expression vector lacking the miR-137 recognition site rescued miR-137-induced precocious differentiation. Furthermore, we demonstrate that TLX, an essential regulator of neural stem cell self-renewal, represses the expression of miR-137 by recruiting LSD1 to the genomic regions of miR-137. Thus, miR-137 forms a feedback regulatory loop with TLX and LSD1 to control the dynamics between neural stem cell proliferation and differentiation during neural development. Stem cells are unique cells with the ability to self-renew and differentiate into multiple cell types. Neural stem cells are a subset of undifferentiated precursors that retain the ability to proliferate, self-renew, and have the capacity to differentiate into both neuronal and glial lineages [1] . Although the functional properties of neural stem cells have been studied extensively, understanding the molecular mechanisms underlying neural stem cell self-renewal and differentiation remains one of the most important tasks in stem cell biology. Accumulating evidence indicates that both transcriptional and post-transcriptional regulations are important mechanisms for regulating genes that are essential for neural stem cell self-renewal and neurogenesis. MicroRNAs (miRNAs) are a recently identified large family of 20–22 nucleotide non-coding RNAs that are involved in numerous cellular processes, including development, proliferation and differentiation [2] , [3] . In the past decade, a network of regulatory circuitries operating at the post-transcriptional level has been uncovered with the finding of a class of miRNA regulators. These molecules have pivotal roles in mediating mRNA stability and translational inhibition of specific target genes [3] . The function of miRNAs has been correlated with many complex cellular functions [2] . While some miRNAs are ubiquitously expressed, others exhibit developmental stage or tissue-specific expression [4] . The study of tissue-specific miRNAs will provide important clues for identifying new regulatory circuitries involved in the control of cell-specific differentiation. Recently, several brain-specific miRNAs have been identified. Among these is miR-137, which has been shown to promote neuronal differentiation of adult subventricular neural stem cells and to inhibit neuronal maturation in adult hippocampal neurons [5] , [6] . However, the role of miR-137 in embryonic brains is still unknown, and the upstream regulators of miR-137 in neural stem cells remain to be identified. TLX (NR2E1) is an orphan nuclear receptor that is expressed in vertebrate forebrains [7] . Mature Tlx knockout mice have significantly reduced cerebral hemispheres, and exhibited increased aggressiveness and progressively violent behaviour [8] , [9] , [10] , [11] . We have shown that TLX is an essential regulator of self-renewal in adult neural stem cell [9] . TLX maintains adult neural stem cells in an undifferentiated and self-renewable state, in part through transcriptional repression of its downstream target genes, such as the cyclin-dependent kinase inhibitor p21 and the tumour suppressor pten, by complexing with histone deacetylases and the lysine-specific histone demethylase lysine-specific demethylase 1 (LSD1) [12] , [13] . In addition to modulation of TLX activity by histone-modifying enzymes, the expression of TLX has been shown to be regulated by miRNAs, including miR-9 and let-7b [14] , [15] . The TLX-positive neural stem cells in the hippocampal dentate gyrus have an important role in spatial learning and memory [16] , whereas the TLX-expressing cells in the subventricular zone of adult brains were shown to be the slowly dividing neural stem cells [17] , [18] , [19] . Recently, we demonstrated that TLX activates the canonical Wnt/β-catenin pathway to stimulate adult neural stem cell proliferation and self-renewal [19] . In addition to its function in adult brains, TLX also has an important role in neural development by regulating cell cycle progression in neural stem cells of the developing brain [20] , [21] , [22] . TLX is therefore a key regulator of neural stem cells in both embryonic and adult brains, although aspects of its downstream events have yet to be uncovered. Epigenetic mechanisms, such as histone modifications, have been shown to have significant roles in the regulation of stem cell proliferation and differentiation [23] . Histone modifications, such as acetylation, phosphorylation and methylation, are switches that alter chromatin structure to form a binding platform for downstream 'effector' proteins to allow transcriptional activation or repression [24] . The recent discovery of a large number of histone demethylases indicates that demethylases have a central role in the regulation of histone methylation dynamics [25] , [26] , [27] , [28] . The first lysyl demethylase identified is LSD1, which demethylates H3K4 or H3K9 in a reaction employing flavin as a cofactor. LSD1 is limited to mono- or dimethylated substrates [26] . We have previously shown that the histone demethylase LSD1 is expressed in neural stem cells and has an important role in neural stem cell proliferation by modulating TLX signalling [13] . LSD1 is recruited to the promoters of TLX downstream target genes to repress their expression, consequently promoting neural stem cell proliferation. However, the upstream events that regulate LSD1 expression remain largely unknown. In this study, we identified miR-137 as a new target of TLX and a novel upstream regulator of LSD1. We demonstrate that TLX represses miR-137 expression in neural stem cells by binding to the 5′ and 3′ sequences of miR-137. Remarkably, one of the targets of miR-137 is the TLX transcriptional co-repressor, LSD1, which is shown to be recruited to the genomic region of miR-137 by TLX to inhibit miR-137 expression. miR-137 inhibits LSD1 expression to regulate neural stem cell proliferation and differentiation. Increased expression of miR-137 led to reduced mouse neural stem cell proliferation and accelerated neural differentiation. In utero electroporation of miR-137 into neural stem cells in the ventricular zone of embryonic mouse brains triggered premature differentiation and outward migration of the transfected cells. Moreover, co-electroporation of an LSD1 expression vector lacking the endogenous 3′-UTR rescued the premature differentiation induced by miR-137 overexpression. Our findings point to the regulatory loop formed between miR-137 and TLX/LSD1 as a critical player in the molecular circuitry controlling neural stem cell proliferation and differentiation during neural development. miR-137 regulates cell proliferation and differentiation The study of tissue-specific miRNAs is important for identifying new regulatory cascades involved in cell fate determination. The brain-enriched miRNA miR-137 is expressed in both embryonic and adult brains. Although the role of miR-137 in adult neurogenesis has been studied [5] , [6] , [29] , its role in neural development remains to be investigated. We first examined whether miR-137 regulates embryonic neural stem cell proliferation and differentiation. For this purpose, primary embryonic neural stem cells were freshly derived from E14.5 mouse brains and transfected with mature miR-137 RNA duplexes. Cell proliferation was determined by 5-bromodeoxyuridine (BrdU) labelling of dividing cells. Transfection of miR-137 led to a dramatic inhibition of cell proliferation ( Fig. 1a,b ) with minimal cytotoxicity ( Fig. 1c ). 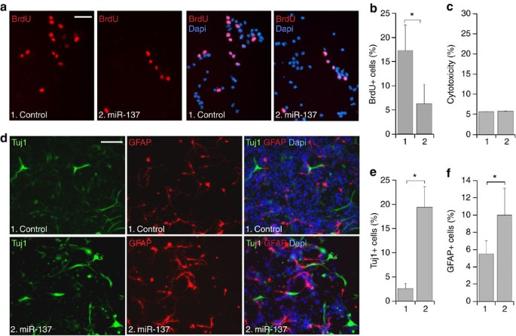Figure 1: Overexpression of miR-137 regulates neural stem cell proliferation and differentiation. (a) Cell proliferation in miR-137-transfected embryonic neural stem cells as revealed by BrdU labelling (red). Right panels show BrdU staining along with 4,6-diamidino-2-phenylindole (DAPI) counter staining. Scale bar, 50 μm. (b) Quantification of BrdU-positive (BrdU+) cells in miR-137-treated neural stem cells with s.d. indicated by error bars. *P<0.001 by Student'st-test.n=7. (c) Minimal cytotoxicity in miR-137-transfected neural stem cells, as revealed by LDH assays for cytotoxicity.n=4. (d) Overexpression of miR-137 promotes neural differentiation. Control RNA or miR-137-transfected cells were induced into differentiation for 5 days, and immunostained with a Tuj1-specific antibody (green) or a GFAP-specific antibody (red). Nuclear DAPI staining is shown in blue. Scale bar, 100 μm. (e) Quantification of Tuj1-positive (Tuj1+) cells in control and miR-137-treated neural stem cells.n=3. (f) Quantification of GFAP-positive (GFAP+) cells.n=3. For both sectionseandf, error bars are s.d. of the mean. *P<0.005 (e), *P<0.1 (f) by Student'st-test. Approximately 4,000 cells were quantified for sectionsb,eandf, respectively. Figure 1: Overexpression of miR-137 regulates neural stem cell proliferation and differentiation. ( a ) Cell proliferation in miR-137-transfected embryonic neural stem cells as revealed by BrdU labelling (red). Right panels show BrdU staining along with 4,6-diamidino-2-phenylindole (DAPI) counter staining. Scale bar, 50 μm. ( b ) Quantification of BrdU-positive (BrdU+) cells in miR-137-treated neural stem cells with s.d. indicated by error bars. * P <0.001 by Student's t -test. n =7. ( c ) Minimal cytotoxicity in miR-137-transfected neural stem cells, as revealed by LDH assays for cytotoxicity. n =4. ( d ) Overexpression of miR-137 promotes neural differentiation. Control RNA or miR-137-transfected cells were induced into differentiation for 5 days, and immunostained with a Tuj1-specific antibody (green) or a GFAP-specific antibody (red). Nuclear DAPI staining is shown in blue. Scale bar, 100 μm. ( e ) Quantification of Tuj1-positive (Tuj1+) cells in control and miR-137-treated neural stem cells. n =3. ( f ) Quantification of GFAP-positive (GFAP+) cells. n =3. For both sections e and f , error bars are s.d. of the mean. * P <0.005 ( e ), * P <0.1 ( f ) by Student's t -test. Approximately 4,000 cells were quantified for sections b , e and f , respectively. Full size image To determine whether overexpression of miR-137 regulates embryonic neural stem cell differentiation, neural stem cells were transfected with control RNA or mature miR-137 RNA duplexes. The transfected cells were induced for differentiation using fetal bovine serum and forskolin. Transfection of miR-137 promoted neuronal differentiation dramatically, leading to a considerable increase in the percent of Tuj1-positive neurons at day 5 of differentiation ( Fig. 1d,e ). Transfection of miR-137 also enhanced astroglial differentiation, although to a lesser extent, with a mild increase in glial fibrillary acidic protein (GFAP)-positive astrocytes ( Fig. 1d,f ). These results indicate that miR-137 accelerates neuronal and glial differentiation of neural stem cells. miR-137 stimulates neuronal differentiation in the brain During development, neural stem cells reside in the ventricular zone and subventricular zone, and migrate out into cortical plate upon differentiation. To determine whether miR-137 influences neural stem cell proliferation and differentiation in embryonic brains, mature miR-137 RNA duplexes were introduced into neural stem cells in the ventricular zone of E13.5 mouse brains by in utero electroporation. Electroporated brains were analysed at E15.5. Cells that had taken up miR-137 were labelled red by co-expression of red fluorescent protein (RFP). Transfection of miR-137 led to a marked decrease of cells that were positively labelled for Ki67, a proliferative marker, as revealed by reduced Ki67+RFP+ cells ( Fig. 2a,c ). A substantial increase in the number of cells that migrated to the cortical plate was also observed in miR-137-electroporated brains ( Fig. 2b,d ). These results suggest that miR-137 negatively regulates neural stem cell proliferation and accelerates neural differentiation. 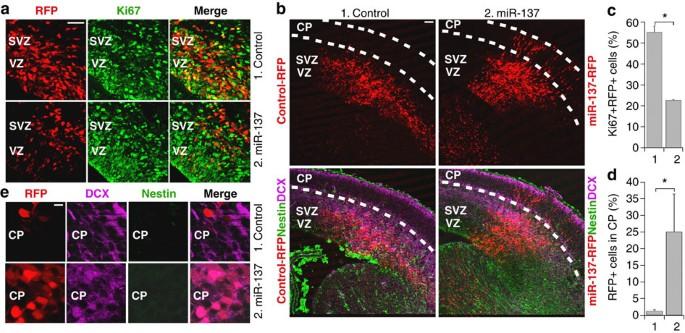Figure 2:In uteroelectroporation of miR-137 in embryonic neural stem cells. (a)In uteroelectroporation of miR-137 decreased cell proliferation in the ventricular zone (VZ) and subventricular zone (SVZ) of embryonic brains. The electroporated cells were RFP+. Proliferating cells were labelled by Ki67. Scale bar, 50 μm. (b) Electroporation of miR-137 led to precocious outward cell migration. The transfected cells were shown red because of the expression of RFP marker. CP, cortical plate. Scale bar, 100 μm. (c) Percentage of Ki67-positive cells out of RFP-positive cells (Ki67+RFP+/RFP+) in miR-137-electroporated brains (2) and control RNA-electroporated brains (1). s.d. is indicated by error bars. *P<0.001 by Student'st-test.n=3. (d) Percentage of control RNA (1) and miR-137 -electroporated cells (2) (RFP+ cells) that migrated to the CP at E15.5 was plotted. Error bars are s.d. of the mean. *P<0.05 by Student'st-test.n=3. (e) Enlarged images of immunostained cells in the CP of control-RFP or miR-137-RFP-electroporated brains collected at E15.5. Scale bar, 10 μm. Figure 2: In utero electroporation of miR-137 in embryonic neural stem cells. ( a ) In utero electroporation of miR-137 decreased cell proliferation in the ventricular zone (VZ) and subventricular zone (SVZ) of embryonic brains. The electroporated cells were RFP+. Proliferating cells were labelled by Ki67. Scale bar, 50 μm. ( b ) Electroporation of miR-137 led to precocious outward cell migration. The transfected cells were shown red because of the expression of RFP marker. CP, cortical plate. Scale bar, 100 μm. ( c ) Percentage of Ki67-positive cells out of RFP-positive cells (Ki67+RFP+/RFP+) in miR-137-electroporated brains (2) and control RNA-electroporated brains (1). s.d. is indicated by error bars. * P <0.001 by Student's t -test. n =3. ( d ) Percentage of control RNA (1) and miR-137 -electroporated cells (2) (RFP+ cells) that migrated to the CP at E15.5 was plotted. Error bars are s.d. of the mean. * P <0.05 by Student's t -test. n =3. ( e ) Enlarged images of immunostained cells in the CP of control-RFP or miR-137-RFP-electroporated brains collected at E15.5. Scale bar, 10 μm. Full size image Neuronal differentiation of the migrated cells was analysed at E15.5 by doublecortin (DCX) staining. Immunostaining revealed that transfection of miR-137 led to enhanced neurogenesis in embryonic brains as shown by increased numbers of RFP+DCX+ neuronal cells at cortical plate, compared with control RNA-electroporated brains ( Fig. 2e ). The cells that migrated out to the cortical plate lost the staining of nestin, a neural progenitor marker ( Fig. 2e ). These results together suggest that miR-137 overexpression promotes neuronal differentiation in embryonic brains. miR-137 represses LSD1 expression by targeting its 3′-UTR Using the TargetScan ( www.targetscan.org ) [30] algorithms, miR-137 was predicted to have a conserved target site in the 3′-UTR of the histone demethylase LSD1. This LSD1 target site is conserved in human, mouse, rat and dog ( Fig. 3a ). To validate whether miR-137 targets LSD1, we made a luciferase reporter construct with mouse 227-bp LSD1 3′-UTR containing the predicted miR-137 target site and flanking sequences. The LSD1 3′-UTR sequences were inserted into the 3′-UTR of a Renilla luciferase reporter gene in a siCHECK vector. The RNA duplexes of mature miR-137 were transfected into human embryonic kidney HEK 293 cells along with the corresponding reporter gene. Repression of the reporter gene was observed in miR-137-treated cells ( Fig. 3b ). To test whether the predicted miR-137 target site in the LSD1 3′-UTR is critical for repression of LSD1 expression by miR-137, point mutations disrupting the base pairing between the miRNA and its target gene in the predicted miR-137 target site were introduced into the LSD1 3′-UTR in the luciferase reporter construct. Mutation of the miR-137 target site abolished the repression by miR-137 ( Fig. 3b ). These results indicate that miR-137 represses LSD1 expression through the predicted target site in the LSD1 3′-UTR. 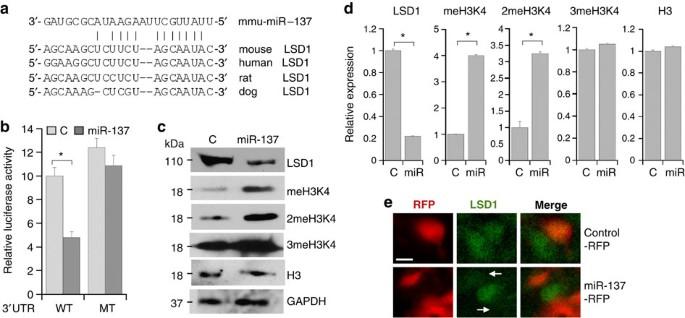Figure 3: miR-137 inhibits LSD1 expression. (a) The nucleotide pairing of miR-137 and LSD1 3′-UTR. (b) miR-137 represses luciferase reporter gene upstream of the LSD1 3′-UTR. Luciferase reporter gene under the control of wild-type (WT) or mutant (MT) LSD1 3′-UTR was transfected along with control RNA (C) or miR-137 RNA duplexes into HEK 293 cells. s.d. is indicated by error bars. *P<0.005 by Student'st-test.n=3. (c) Western blot analysis of LSD1 and methylated histone H3K4 expression in control RNA (C) or miR-137-transfected neural stem cells. Histone H3 (H3) and GAPDH were included as controls. The molecular weight of each band is indicated at the left. (d)Quantification of the western blot results in panelc. The expression of each protein was normalized to the expression of GAPDH. miR stands for miR-137. *P<0.001 by Student'st-test.n=3. (e) Knockdown of LSD1 expression in miR-137-electroporated brains. E13.5 mouse brains werein uteroelectroporated with control RNA-RFP or miR-137-RFP. LSD1 expression was detected by immunostaining shown in green. Arrows indicate miR-137-electroporated cells exhibiting LSD1 knockdown. Scale bar, 10 μm. Figure 3: miR-137 inhibits LSD1 expression. ( a ) The nucleotide pairing of miR-137 and LSD1 3′-UTR. ( b ) miR-137 represses luciferase reporter gene upstream of the LSD1 3′-UTR. Luciferase reporter gene under the control of wild-type (WT) or mutant (MT) LSD1 3′-UTR was transfected along with control RNA (C) or miR-137 RNA duplexes into HEK 293 cells. s.d. is indicated by error bars. * P <0.005 by Student's t -test. n =3. ( c ) Western blot analysis of LSD1 and methylated histone H3K4 expression in control RNA (C) or miR-137-transfected neural stem cells. Histone H3 (H3) and GAPDH were included as controls. The molecular weight of each band is indicated at the left. ( d) Quantification of the western blot results in panel c . The expression of each protein was normalized to the expression of GAPDH. miR stands for miR-137. * P <0.001 by Student's t -test. n =3. ( e ) Knockdown of LSD1 expression in miR-137-electroporated brains. E13.5 mouse brains were in utero electroporated with control RNA-RFP or miR-137-RFP. LSD1 expression was detected by immunostaining shown in green. Arrows indicate miR-137-electroporated cells exhibiting LSD1 knockdown. Scale bar, 10 μm. Full size image Next, we tested whether miR-137 targets LSD1 expression in neural stem cells. Mature miR-137 RNA duplexes were transfected into neural stem cells. A control RNA duplex was included in a parallel transfection. LSD1 expression levels in the transfected cells were examined by western blot analysis. Marked reduction of LSD1 protein levels was detected in miR-137-transfected cells ( Fig. 3c,d ), indicating that miR-137 downregulates endogenous LSD1 expression in neural stem cells. LSD1 has been shown to demethylate mono- or dimethylated H3K4 (ref. 26 ). Consistent with decreased expression of LSD1, increased levels of mono- and dimethylated H3K4 were observed in miR-137-transfected cells, although no significant difference in trimethylated H3K4 and total histone H3 levels was detected ( Fig. 3c,d ). To assess the effect on LSD1 expression by miR-137 in vivo , we in utero electroporated miR-137 RNA duplexes and a RFP reporter (miR-137-RFP) into neural stem cells of E13.5 mouse brains, and immunostained brain sections of the electroporated embryos with LSD1-specific antibody. The expression of LSD1 is reduced dramatically in miR-137-RFP-electropoarted cells, compared with control RNA and RFP-electroporated cells ( Fig. 3e ), providing in vivo evidence that miR-137 targets LSD1 expression. LSD1 rescues miR-137-induced precocious migration To determine whether the effect of miR-137 on neuronal differentiation and migration is mediated through LSD1, an expression vector was prepared to co-express LSD1 without its endogenous 3′-UTR and an RFP reporter (LSD1-RFP) under two independent promoters. In utero electroporation of the LSD1 expression vector lacking its 3′-UTR along with miR-137 (miR-137-LSD1-RFP) rescued the decrease in neural stem cell proliferation ( Fig. 4a,c ) and reversed the precocious migration induced by miR-137 overexpression ( Fig. 4b,d ). Quantification of the RFP+ cells revealed a substantial decrease in the number of RFP+ cells that migrated to the cortical plate in miR-137-LSD1-RFP-electroporated brains, compared with the miR-137-RFP-electroporated brains ( Fig. 4d ). 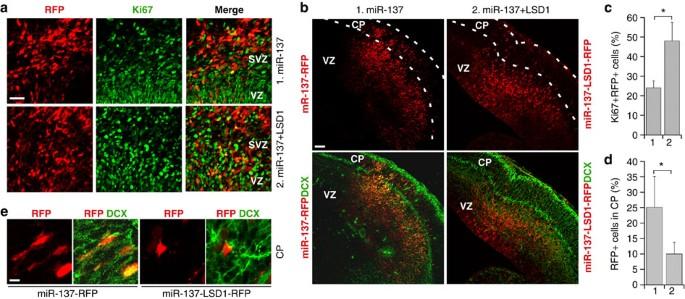Figure 4: Co-transfection of LSD1 without its 3′-UTR rescues miR-137-induced precocious outward migration. (a)In uteroelectroporation of a LSD1 vector without its 3′-UTR along with miR-137 (miR-137+LSD 1) rescued miR-137-mediated decrease in cell proliferation in the ventricular zone (VZ) and subventricular zone (SVZ) of embryonic mouse brains. The electroporated cells were RFP+. Proliferating cells were labelled by Ki67. Scale bar, 50 μm. (b) Electroporation of miR-137 and LSD1 led to rescue of miR-137-induced precocious outward cell migration. The transfected cells were shown red because of the expression of RFP marker. Merged images of RFP and DCX staining were shown at the bottom. VZ, ventricular zone. Scale bar, 100 μm. (c) Percentage of Ki67-positive cells out of RFP-positive cells (Ki67+RFP+/RFP+) in miR-137- and LSD1-electroporated brains (2) and miR-137-alone-electroporated brains (1). s.d. is indicated by error bars. *P<0.05 by Student'st-test.n=3. (d) Quantification of RFP-positive (RFP+) cells that were migrated to the CP. Error bars are s.d. of the mean. *P<0.05 by Student'st-test.n=3. (e) Enlarged images of immunostaining of miR-137-RFP- or miR-137-LSD1-RFP-electroporated brain sections. CP, cortical plate. Scale bar, 10 μm. Figure 4: Co-transfection of LSD1 without its 3′-UTR rescues miR-137-induced precocious outward migration. ( a ) In utero electroporation of a LSD1 vector without its 3′-UTR along with miR-137 (miR-137+LSD 1) rescued miR-137-mediated decrease in cell proliferation in the ventricular zone (VZ) and subventricular zone (SVZ) of embryonic mouse brains. The electroporated cells were RFP+. Proliferating cells were labelled by Ki67. Scale bar, 50 μm. ( b ) Electroporation of miR-137 and LSD1 led to rescue of miR-137-induced precocious outward cell migration. The transfected cells were shown red because of the expression of RFP marker. Merged images of RFP and DCX staining were shown at the bottom. VZ, ventricular zone. Scale bar, 100 μm. ( c ) Percentage of Ki67-positive cells out of RFP-positive cells (Ki67+RFP+/RFP+) in miR-137- and LSD1-electroporated brains (2) and miR-137-alone-electroporated brains (1). s.d. is indicated by error bars. * P <0.05 by Student's t -test. n =3. ( d ) Quantification of RFP-positive (RFP+) cells that were migrated to the CP. Error bars are s.d. of the mean. * P <0.05 by Student's t -test. n =3. ( e ) Enlarged images of immunostaining of miR-137-RFP- or miR-137-LSD1-RFP-electroporated brain sections. CP, cortical plate. Scale bar, 10 μm. Full size image Neuronal differentiation of the migrated cells was analysed by DCX staining. The immunostaining results indicated that electroporation of the expression vector of LSD1 lacking its 3′-UTR along with miR-137 (miR-137-LSD1-RFP) substantially reversed the precocious neuronal differentiation induced by miR-137, as revealed by the decreased numbers of RFP+DCX+ neurons at the cortical plate of miR-137-LSD1-RFP-electroporated brains compared with that of miR-137-RFP-electroporated brains ( Fig. 4e ). In addition to deletion of the entire LSD1 3′-UTR, we also mutated the specific miR-137 target site in the LSD1 3′-UTR. A similar rescue effect on neural stem cell proliferation was achieved by co-electroporation of miR-137 with the LSD1 expression vector harbouring the mutated miR-137 target site in its 3′-UTR, whereas the LSD1 expression vector containing the intact miR-137 target site in its 3′-UTR had minimal rescue effect on neural stem cell proliferation ( Figs 4a,c and 5a,b ). Co-transfection of the LSD1 expression vector with the mutated miR-137 target site also reversed miR-137-induced outward migration ( Figs 4b,d and 5c,d ). These results strongly suggest that miR-137 regulates neural stem cell proliferation and differentiation in embryonic brains through targeting LSD1 expression by base pairing to its 3′-UTR. 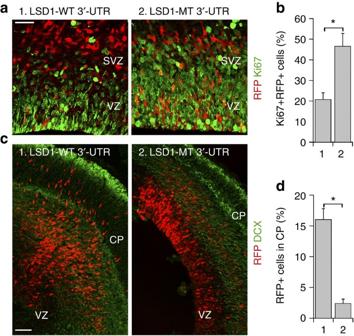Figure 5: Mutation of LSD1 3′-UTR rescues miR-137-induced proliferative defect and precocious migration. (a)In uteroelectroporation of a LSD1 vector with its wild-type 3′-UTR (LSD1-WT 3′-UTR, 1) or mutant 3′-UTR (LSD1-MT 3′-UTR, 2) along with miR-137 into E13.5 mouse brains. The miR-137 + LSD1-MT 3′-UTR treatment, but not miR-137 + LSD1 WT 3′-UTR treatment, increased cell proliferation in the ventricular zone (VZ) and subventricular zone (SVZ) of electroporated brains. The electroporated cells were RFP+. Proliferating cells were labelled by Ki67. Scale bar, 50 μm. (b) Percentage of Ki67-positive cells out of RFP-positive cells (Ki67+RFP+/RFP+) in miR-137 + LSD1-WT 3′-UTR (1)- and miR-137 + LSD1-MT 3′-UTR (2)-electroporated brains. s.d. is indicated by error bars. *P<0.005 by Student'st-test.n=3. (c) Electroporation of miR-137 + LSD1-MT 3′-UTR led to significantly less outward cell migration. The electroporated cells were shown red because of the expression of RFP. Merged images of RFP and DCX staining were shown. CP: cortical plate. Scale bar, 100 μm. (d) Quantification of RFP-positive (RFP+) cells that were migrated to the CP. Error bars are s.d. of the mean. *P<0.001 by Student'st-test.n=3. Figure 5: Mutation of LSD1 3′-UTR rescues miR-137-induced proliferative defect and precocious migration. ( a ) In utero electroporation of a LSD1 vector with its wild-type 3′-UTR (LSD1-WT 3′-UTR, 1) or mutant 3′-UTR (LSD1-MT 3′-UTR, 2) along with miR-137 into E13.5 mouse brains. The miR-137 + LSD1-MT 3′-UTR treatment, but not miR-137 + LSD1 WT 3′-UTR treatment, increased cell proliferation in the ventricular zone (VZ) and subventricular zone (SVZ) of electroporated brains. The electroporated cells were RFP+. Proliferating cells were labelled by Ki67. Scale bar, 50 μm. ( b ) Percentage of Ki67-positive cells out of RFP-positive cells (Ki67+RFP+/RFP+) in miR-137 + LSD1-WT 3′-UTR (1)- and miR-137 + LSD1-MT 3′-UTR (2)-electroporated brains. s.d. is indicated by error bars. * P <0.005 by Student's t -test. n =3. ( c ) Electroporation of miR-137 + LSD1-MT 3′-UTR led to significantly less outward cell migration. The electroporated cells were shown red because of the expression of RFP. Merged images of RFP and DCX staining were shown. CP: cortical plate. Scale bar, 100 μm. ( d ) Quantification of RFP-positive (RFP+) cells that were migrated to the CP. Error bars are s.d. of the mean. * P <0.001 by Student's t -test. n =3. Full size image Regulation of miR-137 expression by TLX We have shown earlier that TLX has an important role in embryonic neural stem cells during neural development [22] . Interestingly, miR-137 is dramatically upregulated in TLX small interfering RNA (siRNA)-treated neural stem cells as revealed by real time reverse transcriptase PCR (RT–PCR) analysis ( Fig. 6a ). The increased expression of miR-137 in TLX siRNA-treated neural stem cells suggests that TLX may be a negative regulator of miR-137 expression. To determine whether the regulation of miR-137 expression by TLX occurs at the transcriptional level, we also checked the level of the primary precursor of miR-137 (pri-miR-137) in TLX siRNA-treated neural stem cells. A similar increase in pri-miR-137 level was detected upon TLX knockdown ( Fig. 6a ), suggesting that miR-137 expression could be regulated by TLX at transcriptional level. As LSD1 is a downstream target of miR-137, we also examined the expression levels of LSD1 in TLX siRNA-treated neural stem cells. As expected, decreased LSD1 expression was detected upon TLX knockdown, opposite to the increase expression of miR-137 ( Fig. 6a ). 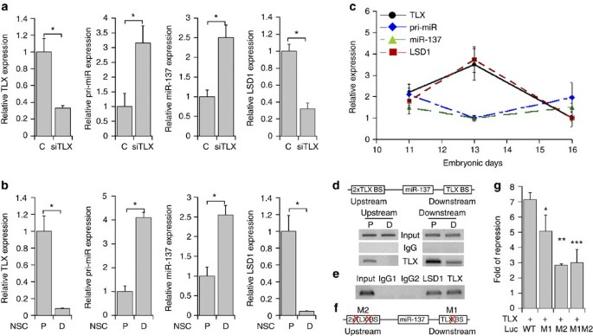Figure 6: TLX regulates miR-137 expression. (a) The expression of TLX, the primary precursor of miR-137 (pri-miR), mature miR-137 and LSD1 in control RNA (C)- and the TLX siRNA (siTLX)-treated embryonic neural stem cells, as revealed by real time RT–PCR analysis. *P<0.001 by Student'st-test.n=3. (b) The expression of TLX, pri-miR, miR-137 and LSD1 in proliferating embryonic neural stem cells (P) and differentiated neural cells (D), as shown by real time RT–PCR. *P<0.001 by Student'st-test.n=3. (c) The expression of TLX, LSD1, pri-miR-137 (pri-miR) and mature miR-137 at E11, E13 and E16, as shown by real time RT-PCR. (d) Binding of TLX to the consensus TLX-binding sites (TLX BS) in miR-137 genomic regions, as revealed by ChIP assays. Two consensus TLX-binding sites are located at miR-137 upstream and downstream genomic regions. ChIP assays were performed using lysates from neural stem cells that were cultured under proliferation (P) or differentiation condition (D). Input: DNA input; IgG: negative control; TLX: pull down with anti-TLX antibody. (e) Recruitment of LSD1 along with TLX to the TLX-binding site in miR-137 genomic region as revealed by ChIP assays. Input: DNA input; IgG1, IgG2: negative controls. (f) Schematic representations of the mutants with mutations (X) in the TLX-binding sites. (g) TLX represses luciferase reporter gene under the control of miR-137 genomic sequences, and mutation of the TLX-binding sites relieves the repression. WT, wild-type TLX-binding sites (TLX BS); M1, mutation of the miR-137 downstream TLX BS; M2, mutation of the miR-137 upstream TLX BS; M1M2, mutation of both miR-137 upstream and downstream TLX BS. *P<0.05; **P<0.001; ***P<0.002 by one-way analysis of variance.n=3. Figure 6: TLX regulates miR-137 expression. ( a ) The expression of TLX, the primary precursor of miR-137 (pri-miR), mature miR-137 and LSD1 in control RNA (C)- and the TLX siRNA (siTLX)-treated embryonic neural stem cells, as revealed by real time RT–PCR analysis. * P <0.001 by Student's t -test. n =3. ( b ) The expression of TLX, pri-miR, miR-137 and LSD1 in proliferating embryonic neural stem cells (P) and differentiated neural cells (D), as shown by real time RT–PCR. * P <0.001 by Student's t -test. n =3. ( c ) The expression of TLX, LSD1, pri-miR-137 (pri-miR) and mature miR-137 at E11, E13 and E16, as shown by real time RT-PCR. ( d ) Binding of TLX to the consensus TLX-binding sites (TLX BS) in miR-137 genomic regions, as revealed by ChIP assays. Two consensus TLX-binding sites are located at miR-137 upstream and downstream genomic regions. ChIP assays were performed using lysates from neural stem cells that were cultured under proliferation (P) or differentiation condition (D). Input: DNA input; IgG: negative control; TLX: pull down with anti-TLX antibody. ( e ) Recruitment of LSD1 along with TLX to the TLX-binding site in miR-137 genomic region as revealed by ChIP assays. Input: DNA input; IgG1, IgG2: negative controls. ( f ) Schematic representations of the mutants with mutations (X) in the TLX-binding sites. ( g ) TLX represses luciferase reporter gene under the control of miR-137 genomic sequences, and mutation of the TLX-binding sites relieves the repression. WT, wild-type TLX-binding sites (TLX BS); M1, mutation of the miR-137 downstream TLX BS; M2, mutation of the miR-137 upstream TLX BS; M1M2, mutation of both miR-137 upstream and downstream TLX BS. * P <0.05; ** P <0.001; *** P <0.002 by one-way analysis of variance. n =3. Full size image Inverse expression profiles of TLX and miR-137 were also observed in neural stem cells under proliferation and differentiation conditions ( Fig. 6b ). While the expression of TLX is relatively high in neural stem cells and reduced upon differentiation, pri-miR-137 and miR-137 expression was induced in differentiated cells ( Fig. 6b ). The expression of LSD1, in turn, was decreased upon differentiation, opposite to increased miR-137 expression ( Fig. 6b ). Furthermore, we examined the expression of TLX, pri-miR-137, mature miR-137 and LSD1 during neural development at E11, E13 and E16. Opposite expression patterns of TLX/LSD1 and miR-137 was observed, with highest expression of TLX and LSD1 at E13, while lower pri-miR-137 and miR-137 expression at E13 ( Fig. 6c ). Sequence analysis revealed three consensus TLX-binding sites in the flanking regions of miR-137 genomic locus, two at the upstream region (located at −1.89 kb and −2.36 kb, respectively) and one at the downstream region (at +630 bp). Chromatin immunoprecipitation (ChIP) analysis revealed that TLX is recruited to both upstream and downstream consensus TLX-binding sites in the miR-137 genomic region in neural stem cells ( Fig. 6d ). Decreased TLX binding was detected when neural stem cells were induced to differentiate. The TLX transcriptional corepressor LSD1 was also detected at the consensus TLX-binding sites in the miR-137 genomic region along with TLX ( Fig. 6e ). To validate the regulation of miR-137 expression by TLX, we cloned the 1.0 kb miR-137 downstream genomic sequences and the 2.56 kb miR-137 upstream genomic sequences that contain the consensus TLX-binding sites and inserted them into the pGL3 basic vector, downstream and upstream of a luciferase reporter gene, respectively. Co-transfection of TLX with the reporter gene in neural stem cells led to sevenfold repression of the reporter activity ( Fig. 6f,g ). Mutation of either the upstream TLX-binding sites (M2) or both upstream and downstream TLX-binding sites (M1M2) substantially relieved the repression. Significant, but relatively mild, relief of repression was also observed when the downstream TLX-binding site (M1) was mutated alone ( Fig. 6f,g ). These results suggest that TLX represses miR-137 expression by binding to the consensus TLX-binding sites in both upstream and downstream genomic sequences of miR-137. We have previously shown that knockdown of TLX expression in embryonic brains by in utero electroporation of a TLX siRNA led to induced neural differentiation as revealed by precocious outward migration of the transfected cells [22] . We show here that TLX represses miR-137 expression ( Fig. 6 ). If miR-137 is an important downstream target of TLX in embryonic brains, we expect that the inhibition of miR-137 activity may rescue the accelerated cell migration induced by TLX siRNA knockdown. For this purpose, we first tested the effect of a miR-137 inhibitor in reporter assays. While transfection of miR-137 led to significant suppression of a luciferase reporter gene upstream of the LSD1 3′-UTR, treatment of the miR-137 inhibitor abolished the inhibitory effect completely ( Fig. 7a ). In contrast, treatment of the miR-137 inhibitor had no effect on let-7b-mediated inhibition of a reporter upstream of the 3′-UTR of its target, TLX ( Fig. 7b ). These results suggest that the miR-137 inhibitor target miR-137 specifically. 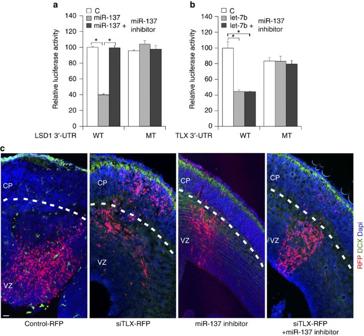Figure 7: A miR-137 inhibitor rescues TLX siRNA-induced outward cell migration in embryonic mouse brains. (a) Treatment with a miR-137 inhibitor abolished the inhibitory effect of miR-137 on the LSD1 3′-UTR reporter. Luciferase assays in cells transfected with a luciferase reporter gene upstream of wild-type (WT) or mutant (MT) LSD1 3′-UTR, along with control RNA (C), miR-137 RNA duplexes or miR-137 RNA duplexes plus the miR-137 inhibitor. (b) Treatment with a miR-137 inhibitor had no effect on the inhibitory effect of let-7b on the TLX 3′-UTR reporter. Error bars are s.d. of the mean. *P<0.001 by Student'st-test, andn=3 for both panelsaandb. (c) Electroporation of control RNA along with a RFP reporter (control-RFP), TLX siRNA with RFP (siTLX-RFP), miR-137 inhibitor with RFP (miR-137 inhibitor) or siTLX-RFP along with the miR-137 inhibitor into E14.5 mouse brains. Migration of the electroporated cells was visualized by RFP fluorescence. VZ: ventricular zone; CP: cortical plate. Scale bar, 100 μm. Figure 7: A miR-137 inhibitor rescues TLX siRNA-induced outward cell migration in embryonic mouse brains. ( a ) Treatment with a miR-137 inhibitor abolished the inhibitory effect of miR-137 on the LSD1 3′-UTR reporter. Luciferase assays in cells transfected with a luciferase reporter gene upstream of wild-type (WT) or mutant (MT) LSD1 3′-UTR, along with control RNA (C), miR-137 RNA duplexes or miR-137 RNA duplexes plus the miR-137 inhibitor. ( b ) Treatment with a miR-137 inhibitor had no effect on the inhibitory effect of let-7b on the TLX 3′-UTR reporter. Error bars are s.d. of the mean. * P <0.001 by Student's t -test, and n =3 for both panels a and b . ( c ) Electroporation of control RNA along with a RFP reporter (control-RFP), TLX siRNA with RFP (siTLX-RFP), miR-137 inhibitor with RFP (miR-137 inhibitor) or siTLX-RFP along with the miR-137 inhibitor into E14.5 mouse brains. Migration of the electroporated cells was visualized by RFP fluorescence. VZ: ventricular zone; CP: cortical plate. Scale bar, 100 μm. Full size image Next, we performed in utero electroporation by co-transfecting the miR-137 inhibitor with a TLX siRNA. While electroporation of the TLX siRNA alone led to precocious cell migration into the cortical plate, co-electroporation of the TLX siRNA with a miR-137 inhibitor led to substantial reverse of the outward migration of the electroporated (RFP+) cells ( Fig. 7c ). This result provides in vivo evidence that miR-137 is an important downstream effector of TLX in embryonic brains. As LSD1 is a target of miR-137, and LSD1 expression was reduced upon TLX siRNA treatment in neural stem cells ( Fig. 6a ), we next tested whether LSD1 overexpression rescues TLX siRNA-induced precocious outward migration. Indeed, co-electroporation of the TLX siRNA with a LSD1 expression vector (LSD1-RFP) reduced the number of cells that migrated to the cortical plate considerably ( Fig. 8 ). 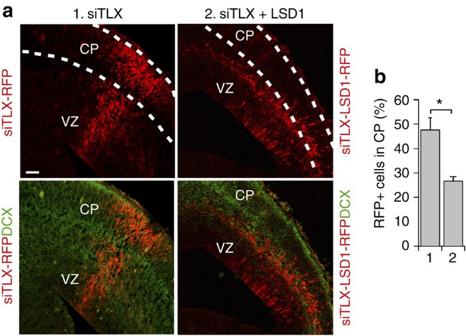Figure 8: LSD1 rescues TLX siRNA-induced outward migration. (a)In uteroelectroporation of a LSD1 vector without its 3′-UTR along with TLX siRNA (siTLX+LSD 1) rescued TLX siRNA (siTLX)-mediated precocious outward migration. The electroporated cells were shown red because of the expression of RFP marker. Merged images of RFP and DCX staining were shown at the bottom. VZ, ventricular zone; CP, cortical plate. Scale bar, 100 μm. (b) Quantification of the RFP-positive (RFP+) cells that were migrated to the CP. Error bars are s.d. of the mean. *P<0.005 by Student'st-test.n=3. Figure 8: LSD1 rescues TLX siRNA-induced outward migration. ( a ) In utero electroporation of a LSD1 vector without its 3′-UTR along with TLX siRNA (siTLX+LSD 1) rescued TLX siRNA (siTLX)-mediated precocious outward migration. The electroporated cells were shown red because of the expression of RFP marker. Merged images of RFP and DCX staining were shown at the bottom. VZ, ventricular zone; CP, cortical plate. Scale bar, 100 μm. ( b ) Quantification of the RFP-positive (RFP+) cells that were migrated to the CP. Error bars are s.d. of the mean. * P <0.005 by Student's t -test. n =3. Full size image In summary, this study allowed us to identify TLX as an upstream regulator of miR-137 expression and LSD1 as a downstream effector of miR-137 action in embryonic brains. The regulatory cascade of TLX-miR-137-LSD1 provides a critical control for embryonic neural stem cell proliferation, differentiation and migration. This study provides the first evidence for the role of miRNA miR-137 in neural development, and identified the lysine-specific histone demethylase LSD1 as a novel miR-137 downstream target. Furthermore, we identified TLX as an upstream regulator of miR-137 expression. We show here that miR-137 forms a regulatory loop with TLX and its transcriptional co-repressor LSD1 to regulate neural stem cell proliferation and differentiation in embryonic brains. TLX and LSD1 are both highly expressed in neural stem cells but repressed upon differentiation [9] , [13] , whereas the level of miR-137 is increased upon differentiation [5] , [29] , [31] . Consistent with the opposite expression pattern of miR-137 and TLX/LSD1, we show that TLX represses miR-137 expression through the recruitment of transcriptional corepressor LSD1. On the other hand, miR-137 suppresses LSD1 expression. This study demonstrates that miR-137 has an important role in embryonic neural stem cell proliferation and differentiation during neural development. Overexpression of miR-137 in embryonic neural stem cells lead to reduced neural stem cell proliferation, as well as enhanced neuronal and glial differentiation. This result is consistent with a previous study showing that transfection of miR-137 promoted neuronal differentiation of adult subventricular zone-derived neural stem cells [5] , although no effect on astrocyte differentiation was detected in the previous study [5] . Interestingly, in a separate study, miR-137 was shown to promote the proliferation and inhibit differentiation of adult hippocampal neural stem cells [29] . These results suggest that the function of miR-137 in neural stem cells could be cellular context-dependent. The important role of miR-137 in embryonic brains established in this study, along with its function in adult neural stem cell proliferation and differentiation described in previous studies [5] , [29] , provides strong evidence that miR-137 is an essential regulator of neurogenesis during multiple developmental stages. Every miRNA may have multiple target genes [30] , [32] . In this study, we identified LSD1 as a key target of miR-137 in neural stem cells of embryonic brains. Several other target genes have also been predicted and/or confirmed for miR-137, including CDK6, a regulator of the cell cycle and differentiation [5] , Ezh2, a histone methyltransferase [29] , and Jarid1b, a histone H3 lysine 4 demethylase [33] . One of the questions addressed here is whether the cell proliferation and differentiation effect mediated by miR-137 in embryonic neural stem cells is directly related to repression of LSD1 expression. Transfection of miR-137 along with an LSD1-expressing vector lacking the miR-137 target site into embryonic neural stem cells in E13.5 mouse brains revealed that expression of LSD1 reversed miR-137-induced precocious differentiation. The result of this rescue experiment suggests that miR-137 regulates neural differentiation in embryonic brains through repression of LSD1 expression. Through regulation of LSD1 (and probably other critical factors), miR-137 seems to regulate multiple aspects of neurogenesis, including neural stem cell proliferation, neuronal and glial differentiation, and neuronal migration. This type of regulation might be common during development in order to control critical signalling pathways and allow proper decisions regarding cell fate transition, cell proliferation and differentiation. Study of miR-137 expression uncovered an interesting regulatory loop involving two established stem cell regulators, the nuclear receptor TLX and its transcriptional co-repressor LSD1. TLX was shown to recruit LSD1 to the miR-137 genomic regions to repress miR-137 primary precursor expression in neural stem cells. In cascade, miR-137 acts by repressing LSD1 expression, thus removing it from the regulatory region of miR-137 genomic loci to maintain sustained levels of miR-137 expression to ensure neural differentiation. These findings are in agreement with the roles described for TLX and LSD1, both of which have been implicated in maintaining and promoting neural stem cell proliferation [9] , [13] . We have shown previously that miRNA miR-9 forms a negative feedback loop with TLX to control neural stem cell fate determination [15] . The regulatory circuitry described here provides another example of how gene regulation during cell differentiation relies on miRNA-mediated tweaking of gene expression. It is also interesting to note that the fine tuning of miR-137 expression is part of a regulatory loop in which repression of the miRNA target gene LSD1 allows for sustained miRNA expression during neural differentiation. In conclusion, our study provides new insights into the molecular processes required for neural differentiation by uncovering a novel regulatory loop between miR-137 and TLX/LSD1. This regulatory circuitry may represent a general mechanism to sense the intricate balance between cell proliferation and differentiation and to allow cell fate determination in a timely manner during development. This study also offers the possibility of identifying new small RNA molecules for the development of novel therapeutic approaches to neurological diseases. Neural stem cell culture and differentiation For embryonic neural stem cell preparation, E14. 5 embryonic brains were collected and meninges were removed. The resultant tissues were dissociated by gentle pipetting. Neural stem cells were prepared by culturing the dissociated cells in polyornithine- and fibronectin-coated plates using N2 medium (DMEM/F12, 25 μg ml −1 insulin, 100 ngml −1 apo-transferrin, 30 nM sodium selenite, 20 nM progesterone and 100 μM putrescine), supplemented with 10 ngml −1 FGF2. For differentiation, embryonic neural stem cells were dissociated into single cells using accutase, and plated on polyornithine and fibronectin-coated plates in N2 medium supplemented with 0.5% fetal bovine serum and 10 μM Forskolin. Cells were allowed to differentiate for 5 days, followed by immuostaining for neuronal and glial markers. For miR-137 treatment-coupled differentiation, cells were first transfected with miR-137, then changed to neural differentiation media 8 h later and kept in this media for 5 days. Transfection and reporter assays Plasmid DNA and DNA–RNA mix were transfected using Transfectin (Bio-Rad). For transfection of RNA duplexes, 20 nM final concentration of miRIDIAN miR-137 mimic (Dharmacon, C-310413-05-005) was mixed with 1 μl DharmaFECT 1 in 20 μl serum-free media, incubated at room temperature for 20 min, and added dropwise to cells in 24-well plates with 450 μl medium to a total volume of 500 μl. The transfected cells were collected 48 h after transfection and subjected to subsequent analyses. The wild-type miR-137 RNA duplex sense sequence is 5′-UUAUUGCUUAAGAAUACGCGUAG-3′. The control RNA duplex sense sequence is 5′-UCACAACCUCCUAGAAAGAGUAGA-3′. We measured Renilla luciferase activity 48 h after transfection, normalized it with firefly luciferase internal control, and expressed it as relative luciferase activity. Western blot analysis Western blot of LSD1, meH3K4, 2meH3K4, 3meH3K4, H3 and glyceraldehyde-3-phosphate dehydrogenase (GAPDH) was performed using anti-LSD1 antibody (Cell Signaling, 1:1,000), anti-meH3K4 (Abcam, 1:1,000), anti-2meH3K4 (Abcam, 1:1,000), anti-3meH3K4 (Abcam, 1:1,000), anti-H3 (Cell Signaling, 1:1,000) and anti-GAPDH antibody (Santa Cruz, 1:1,000). Quantification of western blot was performed using Image J software. RT–PCR analysis Total RNAs were isolated from embryonic mouse brains. Total RNA of 1 μg was used for cDNA synthesis primed by random hexamer. The mature miR-137 expression was quantified by real-time RT–PCR with TaqMan MicroRNA Assays kit for mmu-miR137 (ID 001129, Applied Biosystems). Mouse SnoRNA 202 was used as the internal control (ID 001232, Applied Biosystems). Real-time RT–PCR for primary precursor of miR137 (pri-miR-137), TLX and LSD1 was performed using SYBR Green PCR master mix (Bio-Rad) and StepOnePlus' system (Applied Biosystem). Actin was used as the normalization control. Primers for RT–PCR include pri-miR-137 forward: 5′-TGACAGCGGTAGCAGAGGCAGAG-3′, and pri-miR-137 reverse: 5′-CCGCTGCCCGCCTGCCGCTGGTA-3′; TLX forward: 5′-GGTTCAGACAGCTCCGATTAGAC-3′, and TLX reverse: 5′-TGGAGAGCGGCAATGGCGGCAGC-3′; LSD1 forward: 5′-GGTTTGACTTGTGGAACGTGTGT-3′, and LSD1 reverse: 5′-TGGAAGCCACCTGACAGTAA-3′. BrdU labelling and immunostaining analysis We seeded mouse embryonic neural stem cells at 1x10 5 cells per well in 24-well plates. BrdU was added to cells 48 h after seeding and pulsed for 1–2 h. The BrdU-treated cells were fixed and acid treated, followed by immunostaining analysis with BrdU-specific antibody. Antigen retrieval with sodium citrate buffer (10 mM sodium citrate, pH6.0 and 0.1% Triton X) at 80 °C for 10 min was performed before Ki67 staining. We performed immunostaining using antibodies to BrdU (Accurate, 1:5,000), Ki67 (Thermo Scientific, 1:500), Nestin (Pharmingen, 1:1,000), Tuj1 (Covance, 1:6,000), DCX (Santa Cruz, 1:300) and GFAP (Sigma, 1:1,000). In utero electroporation We performed all animal experiments in accordance with City of Hope and National Institutes of Health guidelines and regulations. For in utero electroporation, mice at 13.5-day gestation were anesthetized with an intraperitoneal injection of ketamine (120 mg kg −1 ) and xylazine (10 mg kg −1 ). The uterine horns were exposed. Plasmid DNA and small RNA mixtures were microinjected through the uterus into the lateral ventricles of embryos by pulled glass capillaries (Drummond Scientific). Electroporation was accomplished by holding the injected brain through uterus with forcep-type electrodes CY650-P5 (Protech International) and delivering square electric pulses (5 pulses, duration 50 ms each, interval 950 ms) to the embryos using electroporator CUY-21 (Protech International). The electroporated mice were killed after 2 days. Brains of embryos were collected and analysed. For neuronal differentiation and migration analyses, we injected 37.5 pmol of miR-137 or control RNA duplexes into the lateral ventricles of E13.5 mouse embryos along with 0.625 μg of pEF-pUb-RFP reporter plasmid using electroporator CUY-21. The electroporated mice were killed after 2 days. For LSD1 rescue experiment, in utero electroporation was performed by injecting 37.5 pmol of miR-137 RNA duplexes mixed with 0.625 μg of pEF-pUb-RFP or pEF-LSD1-pUb-RFP plasmid DNA into the lateral ventricles of E13.5 mouse embryos. The electroporated mice were killed after 2 days. In addition, in utero electroporation was also performed by injecting 37.5 pmol of miR-137 RNA duplexes mixed with 0.625 μg of pEF-LSD1 (with wild-type 3′-UTR)-pUb-RFP (LSD1-WT 3′-UTR) or pEF-LSD1 (with mutant 3′-UTR)-pUb-RFP (LSD1-MT 3′-UTR) plasmid DNA into the lateral ventricles of E13.5 mouse embryos. The WT LSD1 3′-UTR contains mouse LSD1 3′-UTR (2,698–2,925 bp). The MT LSD1 3′-UTR has the wild-type miR-137 target site 5′-AACCAAAG-3′ mutated into 5′-TTGGTTTC-3′. For miR-137 inhibitor rescue experiment, in utero electroporation was performed by injecting 37.5 pmol of TLX siRNA (Dharmacon, J-065577-12-0010), miRIDIAN miR-137 hairpin inhibitor (Dharmacon, IH-310413-07-0005), or the combination of both into the lateral ventricles of E13.5 mouse embryos along with 2 μg of pEF-RFP reporter plasmid. Injection of 37.5 pmol of control RNA along with 2 μg of pEF-RFP reporter plasmid was included as a negative control. The electrophorated mice were killed after 2–3 days. For LSD1 rescue of TLX siRNA treatment experiment, in utero electroporation was performed by injecting 37.5 pmol of TLX siRNA mixed with 0.625 μg of pEF-LSD1. Reporter construct preparation For LSD1 3′-UTR reporter construct, we subcloned DNA fragments encoding mouse LSD1 3′-UTR (2,698–2,925 bp) into siCHECK vector (Promega) to make the LSD1 3′-UTR–siCHECK construct. We mutated miR-137 target site in LSD1 3′-UTR–siCHECK vector by site-directed mutagenesis. The wild-type miR-137 target site 5′-AACCAAAG-3′ was mutated into 5′-TTGGTTTC-3′. To make miR-137 reporter construct, we inserted about 1.0 kb mouse miR-137 downstream genomic sequences (+80 to +1054 bp, with transcription start site as +1) and 2.56 kb miR-137 upstream genomic sequences (−2562 to +1 bp), which contain the consensus TLX-binding sites into pGL3 basic vector (Promega) downstream and upstream of a luciferase reporter gene, respectively. The miR-137 mutant reporter construct has the upstream and/or downstream consensus TLX-binding site AAGTCA mutated to AGATCA by sequential site-directed mutagenesis. ChIP assays We performed ChIP assays using the EZ-ChIP kit (Upstate) with precleaned chromatin from 2×10 6 mouse neural stem cells and 5 μg antibody for each ChIP assay. The antibodies used include antibodies for TLX and LSD1. IgG1 and IgG2 were included as negative controls. The primers for ChIP assays include: miR-137 upstream ChIP forward primer: 5′-GAAATCCGACAGCTTAAGGAGGTTTGA-3′; miR-137 upstream ChIP reverse primer: 5′-CATTGCACAGATAGGATTTGATTTACT-3′, miR-137 downstream ChIP forward primer: 5′-AGTTTAGCAGCATCTTTGAGCGCTGA-3′, miR-137 downstream ChIP reverse primer: 5′-CAGAAAGTTCCACCGGGACCCAGC-3′. Cell death analyses Cytotoxicity of miR-137 transfection was determined by measuring the release of the cytosolic enzyme lactate dehydrogenase (LDH) into culture medium upon cell lysis by LDH assay using the CytoTox 96 Non-Radioactive Cytotoxicity Assay kit (Promega) following manufacturer's instruction. Cytotoxicity (%) was expressed as percentage of LDH released into the medium out of total LDH activity. How to cite this article: Sun, G. et al . miR-137 forms a regulatory loop with nuclear receptor TLX and LSD1 in neural stem cells. Nat. Commun. 2:529 doi: 10.1038/ncomms1532 (2011).